Control of magnetohydrodynamic stability by phase space engineering of energetic ions in tokamak plasmas Virtually collisionless magnetic mirror-trapped energetic ion populations often partially stabilize internally driven magnetohydrodynamic disturbances in the magnetosphere and in toroidal laboratory plasma devices such as the tokamak. This results in less frequent but dangerously enlarged plasma reorganization. Unique to the toroidal magnetic configuration are confined 'circulating' energetic particles that are not mirror trapped. Here we show that a newly discovered effect from hybrid kinetic-magnetohydrodynamic theory has been exploited in sophisticated phase space engineering techniques for controlling stability in the tokamak. These theoretical predictions have been confirmed, and the technique successfully applied in the Joint European Torus. Manipulation of auxiliary ion heating systems can create an asymmetry in the distribution of energetic circulating ions in the velocity orientated along magnetic field lines. We show the first experiments in which large sawtooth collapses have been controlled by this technique, and neoclassical tearing modes avoided, in high-performance reactor-relevant plasmas. Performance in tokamak plasmas has improved to such an extent that it is expected that the next generation machine, ITER [1] , presently under construction, will generate fusion power up to ten times the input power required to maintain its nuclear reactivity. Success in ITER, and in present day tokamaks, relies crucially on optimized cross-magnetic field particle and energy confinement, as well as control of magnetohydrodynamic (MHD) instabilities. Perhaps ironically, the confinement properties of tokamaks have become so good that various techniques are now being deployed to deliberately impair confinement locally in space and sometimes temporally, thereby either avoiding, or initiating controlled, destablization of MHD instabilities. Not doing so can lead to delayed but consequently larger perturbations, which in the case of edge-localized modes [2] , [3] can damage the vessel wall, and in the case of core-localized sawteeth [4] can trigger [5] , [6] , [7] globally confinement-limiting, and potentially disruption-causing, neoclassical tearing modes (NTMs) [8] . In tokamaks, it is well known that instabilities are primarily driven by steepening gradients in the current density or the pressure. Additionally, minority energetic ion populations in ITER, including fusion born alpha particles, will have a considerable effect on plasma stability. 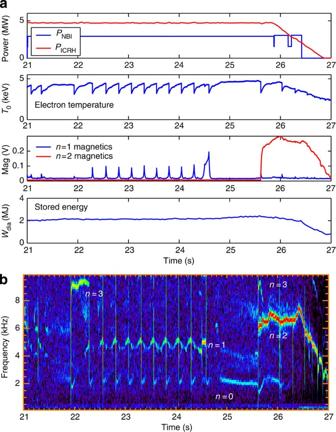Figure 1: JET pulse 78772 in which a long sawtooth period triggers am/n=3/2 NTM despite the pulse being in low-confinement mode. Low concentration3He minority ICRH at around 5 MW is deployed with +90° antenna phasing. This produces co-current propagating waves, thus creating a large tail in the co-passing ion phase space, and long sawteeth. Inathe time traces show the auxiliary power (ICRH power in red and NBI power in blue), the central electron temperature, then=1 (blue) andn=2 (red) magnetics fluctuation amplitudes, and the stored energy. Shown inbis a magnetics spectrogram during the ICRH phase of JET pulse 78772, indicating thatn=1,n=2 andn=3 modes are triggered by consecutive sawtooth crash events. The impact of energetic ions on MHD stability is exemplified in a recent Joint European Torus [9] (JET) pulse 78772, shown in Figure 1 . In this case, the MHD activity can be seen by inspection of the periodic collapse of the core plasma temperature, thus tracing the characteristics of the so-called sawtooth oscillation. In this particular pulse, the energetic ion distributions arising from neutral beam injection (NBI) and ion cyclotron resonance heating (ICRH) were deliberately tuned in order to delay the onset of the sawtooth crash. In this respect, the combined NBI and ICRH simulate the sawtooth stabilizing role of fusion alpha particles in a plasma similar to the standard scenario planned for ITER. In Figure 1a it is seen that following the application of ICRH the longest sawtooth period exceeds one second, which is more than an order of magnitude longer than during the early phase of the pulse without auxiliary heating (the Ohmic phase). Despite the plasma beta (ratio of thermal to magnetic energy) being half that of the expected high confinement mode (H-mode) standard operation in ITER, the magnetics signal indicates the growth of a secondary mode directly following the crash of the long sawtooth. The magnetic island associated with this NTM, with toroidal mode number n =2, is large enough to impair the confinement properties of the plasma, as witnessed by the reduction in the stored energy in Figure 1a . The detection of the NTM by the machine protection system eventually leads to the auxiliary power, current, magnetic field and density being ramped down to avoid a plasma disruption. Figure 1b shows a magnetics spectrogram during the ICRH phase of JET pulse 78772. With exception to the relatively benign n =0 mode [10] , consecutive sawtooth crash events trigger the modes indicated in Figure 1b . In this particular pulse only the n =2 mode becomes a saturated amplitude NTM, but saturation of other n >0 modes can occur, with n =1 typically being the most dangerous. Figure 1: JET pulse 78772 in which a long sawtooth period triggers a m / n =3/2 NTM despite the pulse being in low-confinement mode. Low concentration 3 He minority ICRH at around 5 MW is deployed with +90° antenna phasing. This produces co-current propagating waves, thus creating a large tail in the co-passing ion phase space, and long sawteeth. In a the time traces show the auxiliary power (ICRH power in red and NBI power in blue), the central electron temperature, the n =1 (blue) and n =2 (red) magnetics fluctuation amplitudes, and the stored energy. Shown in b is a magnetics spectrogram during the ICRH phase of JET pulse 78772, indicating that n =1, n =2 and n =3 modes are triggered by consecutive sawtooth crash events. Full size image The traditional method of controlling dangerous MHD activity, such as NTMs, has involved techniques that directly affect the current or pressure gradients in the vicinity of an instability. Such methods enable a degree of control over the timing and amplitude of the MHD oscillation, but are power intensive and would ultimately reduce the reactor's energy efficiency. By contrast, it is shown in this article that instabilities can be controlled effectively without compromising plasma performance by careful tailoring of the phase space properties of auxiliary energetic ion populations. We specialize in the control of the sawtooth instability, and in particular, we demonstrate that the phase space properties of an energetic ion population can be deliberately tuned in the opposite way to those of the JET pulse shown in Figure 1 , so that sawteeth can be shortened in period, and consequential NTMs avoided. This innovative technique, stemming from new theoretical insight, is demonstrated for the first time in high confinement mode (H-mode) plasmas, in which an actuator has created a high-performance reactor-like plasma in quiescent conditions that would otherwise suffer from potentially dangerous NTMs. Energetic ion dynamics in magnetized plasmas Stabilization of MHD modes, by virtually collisionless energetic particles, is not unique to tokamak plasmas. 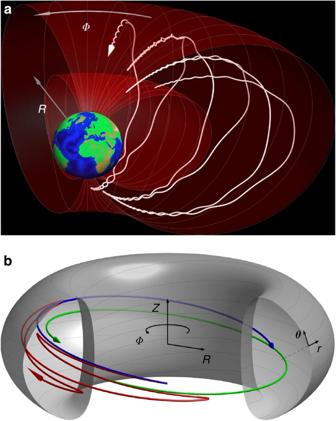Figure 2: Energetic ion orbits confined to the magnetic equilibrium field. The energetic ions in Earth's magnetosphere (a) and the tokamak (b) are confined to spherical and toroidal surfaces, respectively. Three essential types of confined orbits are possible in the tokamak configuration (b) where field lines lie on a toroidal surface: trapped (red), co-passing (blue) and counter-passing (green). Also shown is the toroidal angleφ, along which the dipole and toroidal systems are approximately symmetric, the major radiusR, vertical coordinateZ, poloidal coordinateθand minor radius coordinaterin a torus. Figure 2 compares ion orbits confined in the magnetic field of the earths magnetosphere with ion orbits in the magnetic field lines of the tokamak. The rapid helical gyro motion has been averaged out in the tokamak, so that the guiding centres of particles moving in parallel with, and drifting across, the magnetic field lines can be seen clearly. Hence, the guiding centre velocity with the cross magnetic field drift velocity determined by the non-homogeneity in the magnetic field strength B , and the curvature vector of the magnetic field lines κ . Here, the magnetic moment is an adiabatic invariant over the single particle motion. Magnetically trapped particles occur in both the tokamak and magnetosphere for particles that have sufficiently large pitch μ / ɛ , which is conserved over the particle orbit in a static magnetic equilibrium, where is the kinetic energy of the particle. As a magnetically trapped ion follows the magnetic field lines, it will experience varying B , so that the parallel velocity periodically changes sign and therefore the particle reverses direction, where σ =±1. Such magnetically trapped particle orbits are shown in Figure 2a,b . During the bouncing process along the magnetic field lines, the particle undergoes a cross field drift υ d , resulting in an average precession in the toroidal direction φ . In a tokamak, the toroidal coordinate is an angle of (near) symmetry, as it also is in the magnetosphere assuming a perfect dipole field. The effect of collisional trapped ions on ballooning modes (emerging from transverse Alfvén type waves) and kink modes is destabilizing. Here, a population is considered collisional if particles typically undergo many Coulomb collisions during one bounce cycle. However, the long mean free path kinetic correction associated with near-collisionless trapped ions is stabilizing in both tokamaks [11] , [12] , [13] and the magnetosphere [14] providing that the bounce-averaged drift precession velocity 〈 υ d · e φ 〉 is much larger than the toroidal phase velocity ω /( nR ) of the wave, where a perturbation of the type ∼ exp(− inφ − iωt ) is assumed, R is the distance of the field line from the axis of symmetry as indicated in Figure 2 and e φ is the toroidal unit vector. Figure 2: Energetic ion orbits confined to the magnetic equilibrium field. The energetic ions in Earth's magnetosphere ( a ) and the tokamak ( b ) are confined to spherical and toroidal surfaces, respectively. Three essential types of confined orbits are possible in the tokamak configuration ( b ) where field lines lie on a toroidal surface: trapped (red), co-passing (blue) and counter-passing (green). Also shown is the toroidal angle φ , along which the dipole and toroidal systems are approximately symmetric, the major radius R , vertical coordinate Z , poloidal coordinate θ and minor radius coordinate r in a torus. Full size image Particles that do not undergo bounce trapping are lost to the Earth's atmosphere in Figure 2a . However, in a torus, non-vanishing continuous vector magnetic fields [15] exist, and consequently collisionless untrapped particles can in principle follow magnetic field lines indefinitely without being lost. Such circulating ions are known as co- or counter-passing, with convention defining co-passing as those circulating toroidally in the direction of the (Ohmically induced) toroidal current. This article identifies the crucial effects of collisionless co- and counter-passing particles on general MHD disturbances, including the internal kink mode. The internal kink is a core-localized pressure and current driven mode, whose stability determines the onset of the sawtooth reconnection event, and thus potentially the triggering of an NTM. The novel theoretical advances described here are exploited in the creation of experiments that produce an imbalance in the number, or energy density, of co- and counter circulating ions, and in so doing, control the sawtooth instability in high-performance tokamak conditions. The effect of circulating ions on MHD instabilities In order to assess the impact of collisionless energetic ions on stability, the hybrid kinetic MHD model [16] , [17] is applicable. The linearized equations follow MHD, except that the closure of the system departs from the equation of state, which is only applicable to collisional populations. Breaking the populations into a core (' c ') collisional population and a hot (' h '), essentially collisionless ion population, the linearized equation of motion for components perpendicular to the equilibrium magnetic field B is: where δ denotes a perturbation, P pressure, J current, ρ is the mass density of the majority collisional ion population and ξ is the fluid displacement, obtained in terms of the perturbed electric field via Ohm's law (the parallel perturbed electric field is neglected here), and the hot ion perturbed force density The tensor is obtained by taking moments of the solution δf h of the drift kinetic equation, that is, the Vlasov equation in reduced phase space. The perturbed distribution function about equilibrium f h can be written [18] in terms of perturbations of the three quantities that are conserved in the equilibrium state: where P φ is the toroidal canonical momentum, which is conserved in toroidally symmetric equilibrium. Corrections to the MHD model describing the dynamics of virtually collisionless fast ions are essentially contained in the last term of equation (3), and in a contribution proportional to δ ɛ in the first term of equation (3). In particular, δP φ =−( n / ω ) δɛ − ZeRδA φ , with δA φ the perturbed toroidal magnetic vector potential, and δ ɛ is the change of energy experienced by the particle due to its drift motion across time-varying fields, that is, where the electric field is assumed to be gyro averaged and Ze is the charge of the fast ion. The dynamics associated with δɛ describe the effects of kinetic compressibility, and thus naturally replace the effect of fluid compressibility ordinarily contained in the adiabatic equation of state. 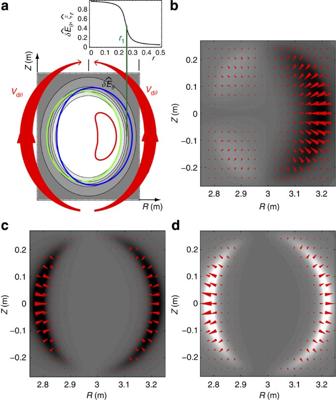Figure 3: The interaction between the fast ions and the internal kink mode instability. Ina, the radial profile of the normalized poloidal electric field, or equivalently the normalized radial fluid displacement, is shown for an internal kink displacement. Also, a contour plot of the poloidal electric fieldacross the poloidal cross-section is shown (a) in conjunction with trapped (red), co-passing (blue) and counter-passing (green)3He ion orbits each with energy 200 keV in toroidal field 3T, together with an illustration of the direction and amplitude of the poloidal drift velocityυdθ.bPlots the radial component of the trapped ion contribution to the response force, whilecanddplot the corresponding contributions due to the radial excursion of, respectively, co- and counter-passing ions. The assumed3He Maxwellian ion population is distributed parabolically in radius. The MHD perturbation takes the form , where in Figure 3 we choose n = m =1, which is appropriate for an internal kink mode displacement associated with the sawtooth instability. Shown in Figure 3a is the radial r component of the normalized unstable internal kink displacement [19] , or the equivalent poloidal electric field in accordance with Ohm's law, as a function of r . The radial component of the perturbed electric field is also important, but for clarity, its effect is not illustrated in what follows. It is seen that varies rapidly at the location r 1 , which is where the parallel wave vector ( nq − m )/ R vanishes, that is, q ( r = r 1 )= m / n , where q measures the pitch d φ /d θ along the magnetic field line. The poloidal electric field in the r — θ poloidal plane is also shown in Figure 3a , with passing and trapped orbits overlaid. The latter are 200-keV 3 He ions orbiting in a 3T tokamak magnetic field. As according to equation (4), the quantity δɛ is a convolution of the drift velocity and the electric field over the guiding centre orbit, the sign (direction) and relative amplitude of the poloidal magnetic drift are also shown. Owing to the fact that trapped ions do not complete a full poloidal circuit, the convolution is dominated by a positive poloidal drift velocity (that is, counter-clockwise in Fig. 3a ). Integrating over velocity space, and assuming that f h is a Maxwellian with 3 He tail temperature 100 keV, parabolically distributed in radius, it is seen in Figure 3b that the radial component of the normalized force points inwards. In the context of the momentum equation (1) this states that the reaction of trapped ions to a radially outward fluid displacement is inwards, that is, the kinetic-trapped ion response attempts to damp the initial perturbation. This effect is responsible for the trapped ion stabilization of low frequency modes in the magnetosphere [14] and the tokamak [12] , [13] . Meanwhile, due to the change of sign in the poloidal drift over the orbit, the effects of circulating ions on δɛ are significant only if the ions observe a large variation in around the poloidal circuit. This occurs especially for particles confined in the region overlapping a resonant MHD surface, and it is in this respect that the mechanism outlined here is relevant to a broad class of modes, including interchange modes [20] , toroidal Alfven eigenmodes [21] and resistive wall modes [22] . For the internal kink mode, counter-passing ions will observe a larger poloidal electric field in the region where the poloidal drift velocity is positive (where the poloidal drift is anti-clockwise in Fig. 3a ), and vice-versa for co-passing ions. This variation in the electric field over the orbit occurs because of the radial drift motion of the single particle across magnetic field lines, as shown in Figure 3a . The radial drift excursion is enhanced as the energy of the single particle is increased relative to a fixed cyclotron frequency. Moreover, circulating particles that are almost trapped have the largest radial drift excursion [23] , and it is these particles that yield the largest contribution to . Finally, it should be noted that there are additional finite orbit width modifications [23] associated with the adiabatic response (the toroidal magnetic potential term) on the right hand side of equation (3), and it is the sum of all the finite orbit width effects that are ultimately evaluated for passing ions. Plotted in Figure 3c,d are the contributions to the radial component of due to the radial excursion of, respectively, co- and counter-passing ions. It is seen that for co-passing particles the force points radially inwards close to r 1 , and thus acts so as to diminish the initial outward plasma displacement. In contrast, counter-passing particles create a force that points radially outward close to r 1 . In this sense, the counter-passing ions have the opposite dynamics to energetic trapped ions, and attempt to amplify the initial outward radial fluid displacement. We note that the forces plotted in Figure 3 have the same normalization, and hence it is seen that passing ion kinetic effects compete with trapped ion kinetic effects. Simulations undertaken with effective tail temperature larger than 100 keV for the same cyclotron frequency show [23] , [24] that passing ion kinetic effects are dominant by virtue of the enhanced radial guiding centre motion. Nevertheless, crucially, we point out here that the effects of co- and counter-passing ions shown in Figure 3c,d almost cancel if the distribution of fast ions is symmetric in the parallel velocity (note that a resonance effect not of concern here can remain under certain conditions [25] ). Figure 3: The interaction between the fast ions and the internal kink mode instability. In a , the radial profile of the normalized poloidal electric field , or equivalently the normalized radial fluid displacement , is shown for an internal kink displacement. Also, a contour plot of the poloidal electric field across the poloidal cross-section is shown ( a ) in conjunction with trapped (red), co-passing (blue) and counter-passing (green) 3 He ion orbits each with energy 200 keV in toroidal field 3T, together with an illustration of the direction and amplitude of the poloidal drift velocity υ d θ . b Plots the radial component of the trapped ion contribution to the response force , while c and d plot the corresponding contributions due to the radial excursion of, respectively, co- and counter-passing ions. The assumed 3 He Maxwellian ion population is distributed parabolically in radius. Full size image Generation of phase space asymmetry in fast ion population It is crucial that sawtooth control is demonstrated in reactor-relevant high-performance conditions. Consequently, the experiments addressed by this paper make the leap to conditions akin to those in ITER, the design of which has been made possible because of our growing understanding of fast ion interaction with sawteeth, as reviewed in refs 26 , 27 . The JET experiments reported here have been designed with large auxiliary heating power, where enhanced co-current NBI power stabilizes sawteeth, and in this respect takes the place of fusion alpha particles in ITER. Sawteeth are controlled by toroidally propagating ion cyclotron resonance frequency (ICRF) waves, with low concentration minority 3 He, as envisaged for the ICRH design in ITER. 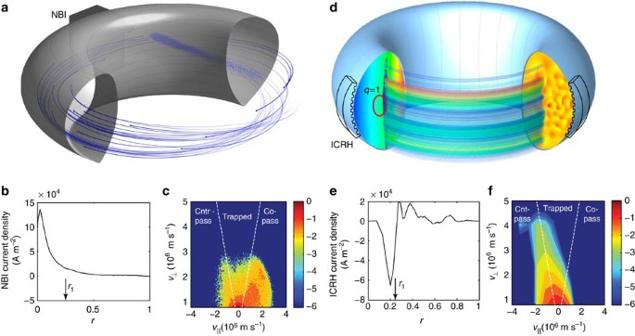Figure 4: The production of energetic ion distribution functions with parallel velocity asymmetry. NBI and ICRH auxiliary heating systems in a JET sawtooth control pulse are shown to yield parallel velocity asymmetry. Inathe NBI system orientation, a simulated particle ionization 'cloud' and ion orbits over 5 μs following NBI switch on. (b)The simulated NBI-driven current plotted with respect to the minor radius normalized to the plasma edge. (c) The distribution of NBI deuterium ions on the low field side close to the rational surfacer1(colour map on logarithmic scale)—see alsoSupplementary Movie 1. Shown in (d) is a sketch of two of the four toroidally spaced A2 ICRH antennas in JET, together with SCENIC code31ICRH simulations: the poloidal cut on the left shows the magnetic field strength, line of ICRH resonance and theq=1 surface. Shown on the right cut is the E-electric field driven by ICRH, while in three dimensions the power deposition is shown through the line of ICRH resonance—see alsoSupplementary Movie 2. Inethe ICRH-driven current is plotted with respect to the minor radius normalized to the plasma edge, and infthe distribution of ICRH ions at the same location, with colour map scaling the same as the NBI distribution inc—see alsoSupplementary Movie 3. In Figure 4, we quantify the degree of asymmetry for auxiliary heating methods used in the JET sawtooth control experiments described below. An illustration of the co-current NBI is shown in Figure 4a , while Figure 4b plots the radial deposition of the current associated with the fast ions. The current is essentially the parallel velocity moment of f h , and is therefore a measure of the degree of parallel velocity asymmetry through the plasma. Figure 4c shows a simulation [28] of the distribution f h of fast ions driven by NBI as a function of the parallel and perpendicular velocity, at a radial location close to the resonant surface r 1 , and a poloidal angle θ =0. As expected for mirror-trapped particles, the distribution is close to symmetric in the trapped cone, while there is a significant asymmetry in the distribution of co- and counter-passing particles. The co-passing particles [23] , [29] and the trapped particles [12] , [13] stabilize the internal kink mode, and therefore sawteeth, by virtue of the mechanism visualized, respectively, in Figure 3b,c . As will be seen, sawteeth are subsequently controlled, or shortened, by depositing 3 He minority ICRH tangent to the internal kink mode resonant surface r 1 on the inboard side of the device, as indicated in the SCENIC code [31] simulations shown in Figure 4d . Counter current propagating waves are employed in order to preferentially heat counter-passing ions. The reason for the extremely effective control on sawteeth is indicated by inspecting the ICRH-driven current density in Figure 4e , where it is seen that very localized asymmetries in the parallel velocity are produced. Figure 4f plots the distribution function of ICRH 3 He ions close to the resonant surface r 1 , where it is seen that a large tail is generated for negative (counter Ohmic current) parallel velocity. Figure 4: The production of energetic ion distribution functions with parallel velocity asymmetry. NBI and ICRH auxiliary heating systems in a JET sawtooth control pulse are shown to yield parallel velocity asymmetry. In a the NBI system orientation, a simulated particle ionization 'cloud' and ion orbits over 5 μs following NBI switch on. ( b )The simulated NBI-driven current plotted with respect to the minor radius normalized to the plasma edge. ( c ) The distribution of NBI deuterium ions on the low field side close to the rational surface r 1 (colour map on logarithmic scale)—see also Supplementary Movie 1 . Shown in ( d ) is a sketch of two of the four toroidally spaced A2 ICRH antennas in JET, together with SCENIC code [31] ICRH simulations: the poloidal cut on the left shows the magnetic field strength, line of ICRH resonance and the q =1 surface. Shown on the right cut is the E-electric field driven by ICRH, while in three dimensions the power deposition is shown through the line of ICRH resonance—see also Supplementary Movie 2 . In e the ICRH-driven current is plotted with respect to the minor radius normalized to the plasma edge, and in f the distribution of ICRH ions at the same location, with colour map scaling the same as the NBI distribution in c —see also Supplementary Movie 3 . 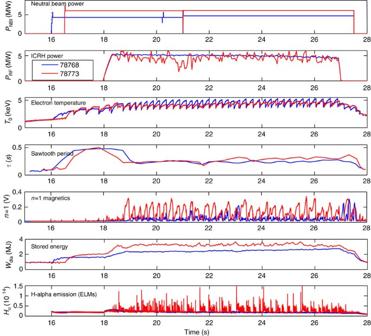Figure 5: Demonstration of sawtooth control and NTM avoidance using ICRH in two high-performance JET pulses. Showing JET pulse 78768 (in blue) with 4.8 MW of NBI and JET pulse 78773 (in red) with 6.4 MW of NBI, where both employed low concentration3He minority ICRH at around 5 MW. In both, the −90° antenna phasing produces counter current propagating waves, which shorten the sawtooth period, shown byτ(s). Also shown is the central electron temperatures in the core, the stored energyWdia, then=1 magnetic perturbation amplitude andHτemission, which indicates that JET pulse 78773 is in high confinement mode. Full size image Sawtooth control in high-performance JET pulses Figure 5 shows JET pulse 78768 in which 4.8 MW of co-current NBI stabilizes the sawteeth, lengthening the period of the initially Ohmic sawteeth of 70 ms to around 500 ms. Following this, a counter-current propagating 33-MHz ICRF wave is generated by the application of ICRH with −90° antenna phasing. The concentration of the ITER-relevant 3 He minority species is about 1%, which has been shown by simulations and JET experiments [24] with relatively low auxiliary heating power, to be the optimum compromise between requiring high-energy minority tail temperature to enlarge the drift orbit excursions (and hence the forces shown in Fig. 3 ), and enabling efficient power transfer between ICRF wave and minority population. With toroidal field 2.9 T and toroidal current 2 MA, the ICRH resonance position is on the inboard (high field side) of the device, lying tangent to the q =1 rational surface. The addition of 5 MW of ICRH in JET pulse 78768 reduces the sawtooth period to around 200 ms despite an increase in energy confinement time (see the stored energy ( W dia ) in Fig. 5 ) and resistive diffusion time due to the increased stored energy and conductivity. Also shown in Figure 5 is the amplitude of the n =1 magnetic field perturbation, driven deliberately large by the application of ICRH, which successfully destabilizes the internal kink mode via the large population of energetic counter-passing ions. In contrast, the long sawtooth JET pulse 78772, shown in the introduction ( Fig. 1 ), employed +90° antenna-phasing ICRH, thereby generating a 3 He distribution with the opposite asymmetry to that shown in Figure 4f , and thus lengthened sawteeth and resultant NTM activity. Meanwhile, in an otherwise similar pulse to 78768, JET pulse 78773 ( Fig. 5 ) begins with a further increased NBI power of 6.4 MW, which once again creates 500-ms sawteeth. The application of 5 MW of ICRH with −90° phasing is sufficient to enhance the auxiliary power above the level required to create a high confinement mode, or H-mode [32] . In this mode of operation, large pressure gradients are created at the plasma edge, which in turn create edge-localized modes, seen by the H α signal in Figure 5 , but have the benefit of raising the density and temperature in the core, as evidenced by the enhancement in the stored energy W dia . These 3 He minority ICRH experiments demonstrate for the first time that sawteeth in H-mode can be efficiently controlled by phase space engineering, where the sawtooth period has been reduced by a factor of two in this case. Such surgical but sustained instability control, by just tailoring the orbits of the energetic ion population, is an optimum solution for ITER or fusion reactors, where fusion energy production would ideally not be compromised by MHD control techniques. Figure 5: Demonstration of sawtooth control and NTM avoidance using ICRH in two high-performance JET pulses. Showing JET pulse 78768 (in blue) with 4.8 MW of NBI and JET pulse 78773 (in red) with 6.4 MW of NBI, where both employed low concentration 3 He minority ICRH at around 5 MW. In both, the −90° antenna phasing produces counter current propagating waves, which shorten the sawtooth period, shown by τ ( s ). Also shown is the central electron temperatures in the core, the stored energy W dia , the n =1 magnetic perturbation amplitude and H τ emission, which indicates that JET pulse 78773 is in high confinement mode. 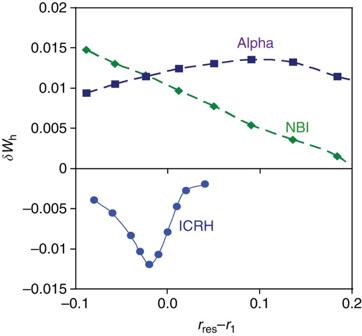Figure 6: Demonstration that the ICRH population in ITER could be tuned to cancel and thereby control the stabilizing effects of alpha particles on the internal kink mode. Plotted are simulations of theδWcontributions to the internal kink mode from alpha particles, neutral beam ions (33MW) and ICRH ions (20MW), assuming 1%3He minority in a standard deuterium-tritium ITER plasma scenario1. These are plotted against the difference between ICRH resonance positionrresand the internal kink mode resonance radiusr1, each normalized to the edge radius. In the simulations,rreswas held constant on the low field side of the device, andr1varied. Full size image Predictions of sawtooth control in ITER using ICRH The simulations shown in Figure 6 predict that the stabilizing effect of fusion alpha particles on sawteeth in ITER could be completely neutralized with 20 MW of low concentration (1%) 3 He minority ICRH in a standard deuterium-tritium ITER plasma scenario [1] . The fast ion mechanism described, and experimentally demonstrated, in this article is quantified in Figure 6 in terms of the potential energy integrated over the plasma volume Figure 6: Demonstration that the ICRH population in ITER could be tuned to cancel and thereby control the stabilizing effects of alpha particles on the internal kink mode. Plotted are simulations of the δW contributions to the internal kink mode from alpha particles, neutral beam ions (33MW) and ICRH ions (20MW), assuming 1% 3 He minority in a standard deuterium-tritium ITER plasma scenario [1] . These are plotted against the difference between ICRH resonance position r res and the internal kink mode resonance radius r 1 , each normalized to the edge radius. In the simulations, r res was held constant on the low field side of the device, and r 1 varied. Full size image where ξ * is the complex conjugate of ξ . The potential energy is obtained in terms of the perturbed force for each fast ion species, as calculated in Figure 6 . The total fast ion potential energy is the sum of these terms. These simulations, obtained from the HAGIS [26] , [33] guiding centre code, demonstrate that while the ITER NBI population (produced from 33MW of 1 MeV neutral particles) and the simulated fusion alpha particle populations are stabilizing (positive δW ) to an internal kink mode displacement in ITER, the ICRH population is strongly destabilizing (negative δW ) providing the ICRH resonance radius r res is sufficiently close to the internal kink mode resonant surface r 1 , and with appropriate phasing of the ICRH antenna. These ITER-dedicated simulations, together with the JET experiments reported here, greatly increase confidence that NTMs and disruptions triggered by sawteeth can be avoided in ITER. Furthermore, additional control techniques [26] , [27] , such as electron cyclotron current drive [34] , could be much more effective in plasmas where ICRH has nullified the stabilizing effects of alpha particles. Minority populations of energetic ions in ITER, including fusion born alpha particles, are expected to have a strong impact on plasma stability. Success in ITER, and in present day tokamaks, relies crucially on the control of MHD instabilities. The deployment of techniques that directly affect the current or pressure gradients in the vicinity of the instability can control the timing and amplitude of MHD oscillations, but such methods are power intensive and would ultimately reduce the reactor's energy efficiency. By contrast, careful tailoring of the phase space properties of auxiliary energetic ion populations will enable MHD instabilities to be controlled effectively without compromising plasma performance. In this article, a mechanism has been identified capable of controlling MHD instabilities by velocity phase space engineering in tokamaks. The mechanism is unique to a toroidally confined plasma, in which energetic particles that are not magnetically bounce trapped can be distributed asymmetrically in the velocity parallel to the magnetic field. Such a population can damp or enhance the growth rates of MHD oscillations ordinarily driven internally by gradients in the plasma pressure. The experiments described here deliberately create such an energetic ion population in order to successfully control crucial core-localized sawteeth, thereby enabling fusion reactor-relevant high-performance tokamak plasmas to be generated free from disruption-limiting NTMs. This permits safe operation at higher plasma pressures and ultimately an improved fusion yield. The JET tokamak In operation since 1983, JET was explicitly designed to study plasma behaviour in conditions and dimensions approaching those required in a fusion reactor. Today, the primary task of JET is to prepare for the construction and operation of ITER. In the core of the machine is the vacuum vessel where the fusion plasma is confined by means of strong magnetic fields and plasma currents (up to 4 T and 5 MA). In the current configuration, the major and minor radii of the plasma torus are R 0 =3 m and r =0.9 m, respectively, and the total plasma volume is up to around 100 m 3 . A divertor at the bottom of the vacuum vessel allows escaping heat and gas to be exhausted in a controlled way. Other features of JET particularly relevant to the experiments described here are a flexible and powerful plasma auxiliary heating system, consisting of NBI, ICRH and lower hybrid current drive. JET also has an extensive diagnostic suite of around 100 individual instruments. JET minority 3 He ICRH experiments As described in the Results, a key objective was to use ITER-relevant minority 3 He for the ICRH. Performing heating with fundamental resonance required that we set the frequency of the ICRH actuators to the minimal value of 33 MHz (28 MHz is possible, but the coupled power efficiency is not optimal). The objective was for the ICRH resonance to be aligned with the q =1 radius, either on the high field side or the low field side. Resonance on the low field side of the device required a prohibitively high toroidal field, so high field side heating resonance was chosen. However, with the fundamental 3 He resonance on the q =1 surface (on the high field side), care had to be taken to ensure that the major radius position of the fundamental hydrogen resonance was larger than the major radius of the ICRH antenna. This set a minimum toroidal magnetic field of around 2.9 T, and a minimum major radius of the q =1 surface on the high field side of 2.75 m. A configuration was chosen that had a large magnetic axis radius ( R 0 ) so that the minor radius of the q =1 surface could be as large as possible despite the restrictions of the ICRH resonance position. This configuration therefore had large inner clearance and a small distance between the antenna and last closed flux surface (thus also aiding ICRH power coupling). A toroidal current of around 2 MA enabled the required q =1 minor radius to be r 1 ≈0.3 m. The optimal conditions for controlling sawteeth were identified in preliminary pulses (not shown in this article). These were obtained by examining the sawtooth period while varying the toroidal magnetic field. During the two pulses shown in Figure 6 , the toroidal magnetic field was ramped very slowly from 2.9 T to 2.96 T, and the toroidal current was ramped proportionally. All the A2 ICRH antennas were employed with −90° antenna phasing (except for the sawtooth stabilizing demonstration pulse shown in Figure 1 where +90° phasing was used). The concentration of the ITER-relevant 3 He minority species was about 1%, which has been shown by simulations and experiments [24] to be optimal for sawtooth control. Such low 3 He concentrations were maintained by minimal opening of the gas valve at the start of the pulse, or by relying on 3 He accumulated on the wall of the machine. Simulations of ICRH fast ion population The SCENIC [31] code was used in this paper to obtain the equilibrium distribution of ICRH ions, as exhibited in, for example, Figure 4d–f . SCENIC was created for integrated modelling of ICRH scenarios in arbitrary fusion plasma geometries. It evolves the MHD equilibrium, dielectric tensor (and thus ICRH wave field propagation and power deposition) and resonant particle species distribution functions in an iterative way. This allows for a self-consistent solution of the plasma state in the presence of a fast wave with prescribed frequency. The final state includes the effects of anisotropic pressure. Even though limited to low-order Larmor radius effects in the dielectric tensor, SCENIC is an efficient tool to investigate 3 He minority heating in a D main plasma, where both mode conversion and second harmonic resonances are negligible. The evolution of the hot particle distribution function is computed with a Monte–Carlo scheme, simulating wave–particle interactions, including Doppler shift and unapproximated wave number. The moments of the distribution function are taken directly from the marker distribution thus incorporating the effects of a non-Maxwellian tail. For the results presented in this work, four million markers have been propagated on 1,024 processors. Steady state has been reached after 12 iterations of 25 ms each, so that the total simulation time is a few collisional slowing down times of the fast ions. Markers were initialized according to a thermal Maxwellian distribution representing the initial state without ICRH, but a weighting scheme was applied in order to achieve more resolution in the tail. Simulations of NBI fast ion population Simulations of the neutral beam slowing down were carried out using an NBI module [28] working in the VENUS guiding centre code described in ref. 31 . The presence of fractional beam energies, beam collimation and multi-step corrections to the ionization cross-section are some of the implemented features. VENUS simulations are run with three million deuterium markers, which is sufficient to represent the crucial characteristics of the NBI population generated from the JET NBI sources. In the numerical scheme, continuous NBI injection is imitated by adding to the simulation 75 subsamples of 4×10 4 markers every t =6.6×10 −3 s. The guiding centre motion is then simulated together with particle slowing down and pitch angle scattering effects, both embedded in a Coulomb collision term. Overall, the numerical run requires 3.2×10 3 CPU hours to accurately describe half a second of NBI at JET. Simulations of fast ion effects on internal kink The effect of the fast ions on the internal kink mode stability is tested using the Monte–Carlo guiding centre drift kinetic code HAGIS [33] . The equilibrium is calculated with a static fixed-boundary two-dimensional Grad–Shafranov solver. The stability of this equilibrium is then tested using a linear MHD stability code. The perturbations from the linear MHD code, and the equilibrium, are then fed into HAGIS together with the distribution functions of fast ions from the ICRH and NBI modules described above (another similar module is used to simulate the alpha particle population). HAGIS is a Monte–Carlo code, which solves the nonlinear drift guiding centre equations of motion. It allows the evolution of a fast ion population to be studied in the presence of electromagnetic perturbations in a toroidal plasma. Calculated here is the perturbed distribution δf h in response to the effect of the internal kink mode perturbation on each of the fast ion populations (ICRH, NBI and alpha particles). We extract δf h during its linear growth phase. Then, we integrate over all phase space for each species to obtain δW h , as defined by equations (2) and (5), where for each species the form of the fast ion pressure tensor is taken to be purely diagonal. When making a scan over r 1 − r res , as in Figure 6 , the marker distributions are unchanged, but the equilibrium q profile is modified (with corresponding new equilibrium and MHD linear stability calculations) in subsequent HAGIS simulations. How to cite this article: Graves, J.P. et al . Control of magnetohydrodynamic stability by phase space engineering of energetic ions in tokamak plasmas. Nat. Commun. 3:624 doi: 10.1038/ncomms1622 (2012).